Hierarchical densification and negative thermal expansion in Ce-based metallic glass under high pressure The polyamorphsim in amorphous materials is one of the most fascinating topics in condensed matter physics. In amorphous metals, the nature of polyamorphic transformation is poorly understood. Here we investigate the structural evolution of a Ce-based metallic glass (MG) with pressure at room temperature (RT) and near the glass transition temperature by synchrotron X-ray diffraction, uncovering novel behaviours. The MG shows hierarchical densification processes at both temperatures, arising from the hierarchy of interatomic interactions. In contrast with a continuous and smooth process for the low- to medium-density amorphous state transformation at RT, a relatively abrupt and discontinuous transformation around 5.5 GPa is observed at 390 K, suggesting a possible weak first-order nature. Furthermore, both positive and abnormal-negative thermal expansion behaviours on medium-range order are observed in different pressure windows, which could be related to the low-energy vibrational motions and relaxation of the weakly linked solute-centred clusters. The microstructure transformations in glasses and liquids induced by high pressure or temperature can substantially alter their dynamical and transport properties [1] , [2] , [3] , [4] , [5] . However, in many respects the nature of pressure- and / or temperature-induced transformation in glasses remains unclear. Since the work of Sheng et al. [6] , it has been realized that polyamorphism is possible in metallic glasses (MGs) despite their non-directional nature of metallic bonds and atom dense-packing characteristic. It was proposed, from ab initio calculation and the genetic isostructural γ–α transition of Ce metal, that the mechanism was due to the pressure-induced 4 f electron delocalization [6] , [7] , [8] . Later on Zeng et al. [9] presented the 4 f electron-delocalization evidence under high pressure from the X-ray absorption spectroscopy experiment. The amorphous-to-amorphous transformation has been also reported in other rare earth element-based MGs (REMGs), suggesting the electronic-structure inheritance of lanthanide-solvent atoms in REMGs [10] , [11] , [12] , [13] , [14] . Nevertheless, at present the nature of the electronic localization–delocalization transition (related to the Kondo volume collapse) is very obscure in these REMGs. And little is known about how the medium-range order (MRO), short-range order (SRO) and free-volume zones react to external pressure, although intensive research has been carried out on the effects of MRO, SRO and free-volume zones on the mechanical and relaxation behaviours in various MGs [15] , [16] , [17] . Furthermore, it is worth noting that the polyamorphic transformation is gradual and occurs in a broad pressure range in all the reported REMGs showing polyamorphism. Accordingly, the existence of a first-order structure transformation in the amorphous metallic system is ambiguous, although distinct polymorphs of REMGs have been recognized recently. It seems that the transformation in REMGs is fundamentally different from the archetypal first-order polyamorphic transformation in amorphous H 2 O, where discontinuous volume change was observed [1] , [18] . Actually, whether the polyamorphic transformation is continuous or truly first order in nature in many amorphous solids remains a strongly debated issue [18] , [19] , [20] , [21] , [22] , [23] , [24] , [25] . In the present letter, the in situ synchrotron X-ray diffraction (XRD) measurements under high pressure on a Ce-based MG both at room temperature (RT) and near (below) the glass transition temperature ( T g ) are carried out comparatively. Ce-based MG is chosen as a model system since its polyamorphsim has been well documented [9] , [10] , [11] , [12] . In addition, the Ce-based MGs possess various attracting properties, such as heavy fermion behaviour, polymer-like thermoplastic performance near RT and anomalous soft longitudinal acoustic mode under high pressure or with decreasing temperature, indicating their unique atomic/electronic structures [26] , [27] , [28] . Here, we report the hierarchical densification processes of amorphous Ce 65 Co 25 Al 10 under high pressure both at RT and near T g , relating to the different degrees of contributions from the weakest atomic configurations, MRO and SRO under different pressure windows. Moreover, a relatively discontinuous change of volume is observed around 5.5 GPa near T g , while only a smooth and continuous change is observed at RT (293 K). The discontinuous change in volume implies a possible first-order-like nature of the polyamorphic transformation, which is hidden thus far in previous experiments due to kinetic sluggishness at lower temperatures. Strikingly, the Ce 65 Co 25 Al 10 MG shows abnormal-negative thermal expansion (NTE) under a pressure range of 0.6–9.0 GPa, which could arise from a combination of the relaxation (minor role) and tilting or rocking motions of the tightly bonded polyhedral clusters linking to weakest atom zones. The relaxation experiments indicate that structure relaxation plays only a minute (secondary) effect on the polyamorphic transformation and the NTE behaviour. Instead, pressure induced bond shorting and local atomic rearrangement, which are assisted significantly from the 4 f electron localization, play the dominate role on the polyamorphic transformations and the abnormal thermal expansion. Structure evolution at RT Synchrotron XRD patterns, obtained in situ as a function of hydrostatic pressure, of the Ce-based MG are shown in Fig. 1a . The sample remains fully amorphous up to the maximum pressure of 50 GPa, as indicated by the halo patterns and absence of sharp Bragg peaks. It is seen from the figure that the first sharp diffuse diffraction peak (FSDP) shifts towards higher Q with increasing pressure due to the compression effect. Besides, the diffraction intensity maxima in the Q regions of 3.0–4.5 Å −1 and 5.0–6.5 Å −1 diminished gradually, whereas those between 4.0 and 5.5 Å −1 intensified with increasing pressure. Significant differences are clearly seen between the XRD patterns recorded at 50 and 0.6 GPa, indicating distinct amorphous phases existing in different pressure ranges. Recently, a pressure-induced devitrification into a single crystal with fixed crystallographic orientation was reported in Ce 75 Al 25 MG [29] . It was argued that the pressure-induced 4 f electron delocalization eliminated the mismatch between Ce and Al atoms and manifested the hidden long-range topological order. Moreover, the pressure-induced devitrification was showed to occur only within a very narrow solute concentration region (19–27% Al for the binary Ce–Al MG) [13] . The preservation of the amorphous structure up to 50 GPa observed here is due to the Co addition in Ce 65 Co 25 Al 10 MG, which enhances both the glass-forming ability and the stability against devitrification under high pressure. Note also that the solute concentration here, 35%, is large enough to fall out of the region where the pressure-induced devitrification can occur [13] . The inset in Fig. 1c is a schematic illustration of the hierarchical amorphous structure of Ce 65 Co 25 Al 10 MG, involving weakly bonded solvent atoms, (Co or Al) solute-centred clusters (SCCs) and superclusters, whose interactions with pressure will be discussed later. 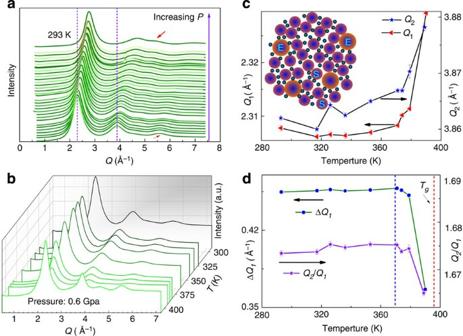Figure 1: Pressure- and temperature-induced structure change. (a)In situXRD patterns of the Ce65Al10Co25MG under high pressure from 0.6 to 50 GPa at RT. (b) XRD patterns at different temperatures under 0.6 GPa. (c) Temperature dependence ofQ1andQ2. The inset is the schematic illustration of a hypothetical amorphous structure of Ce-based MG showing weakly bonded solvent atoms (Ce: the smallest ball), (Co or Al) solute-centred clusters (S) and superclusters (E). The undertint in E and S denotes the outmost shell constituted with a majority of solvent atoms (Ce). (d) Temperature dependence ofQ2/Q1and the full width at half maximum ofQ1. Error bars incanddrepresent the accuracy ofQ1andQ2detemined from the fitting. Figure 1: Pressure- and temperature-induced structure change. ( a ) In situ XRD patterns of the Ce 65 Al 10 Co 25 MG under high pressure from 0.6 to 50 GPa at RT. ( b ) XRD patterns at different temperatures under 0.6 GPa. ( c ) Temperature dependence of Q 1 and Q 2 . The inset is the schematic illustration of a hypothetical amorphous structure of Ce-based MG showing weakly bonded solvent atoms (Ce: the smallest ball), (Co or Al) solute-centred clusters (S) and superclusters (E). The undertint in E and S denotes the outmost shell constituted with a majority of solvent atoms (Ce). ( d ) Temperature dependence of Q 2 / Q 1 and the full width at half maximum of Q 1 . Error bars in c and d represent the accuracy of Q 1 and Q 2 detemined from the fitting. Full size image Thermal expansion below T g under 0.6 Gpa To further explore the structure evolution under high temperature and high pressure, we heated the sample in a diamond anvil cell (DAC) under a constant pressure of 0.6 GPa. When reaching 390 K, we fixed the temperature and increased the pressure to around 42.6 GPa. Figure 1b shows the XRD patterns recorded under a fixed pressure of 0.6 GPa and at different temperatures from RT to 390 K (which is 6 K below the T g ~396 K to ensure that the fully amorphous structure is retained during heating). Normally, the glass transition temperature depends on the external pressure (a increasing pace of 4.4 K GPa −1 has been observed in a Zr-based MG [2] ). Thus, a change (possible increase) of ~3–6 K of T g can be expected under 0.6 GPa, and the temperature-induced supercooled liquid to glass transition process did not occur during our whole investigations. From Fig. 1 , temperature-induced significant atomic change without any crystalline phases can be clearly seen from the changes of intensity and shape of the three maxima between 3.0 and 6.0 Å −1 . Surprisingly, abnormal thermal expansion behaviour in the intermediate-range structure is observed, as illustrated from the temperature dependence of the positions of the first and second maxima ( Q 1 and Q 2 ) of the scattering curves ( Fig. 1c ). The positions of the maxima were calculated by a fit of pseudo-Voigt functions, through which the peak positions can be determined with high accuracy (s.d. σ =±0.002 nm −1 is estimated for the first maximum position at Q 1 ). When the temperature increases from 293 to 317 K, the Q 1 first decreases slightly, through a roughly constant value between 317 and 340 K, then increases gradually above 340 K and accelerates to a rapid pace above 370 K. Similar trend has also been observed for Q 2 . It is generally accepted that the FSDP embodies the MRO feature of various kinds of glasses and its position is inversely proportional to the mean atomic spacing below T g [30] , [31] , [32] , [33] . For MGs a fractal network with a dimension of 2.31 was also reported to describe the MRO by Ma et al. [30] The shift to higher Q with increasing temperature indicates that the characteristic distance in real space was reduced. This behaviour is totally different from those of the Cu- and Pd-based MGs under ambient pressure, where the Q 1 decreases with increasing temperature continuously until the crystallization temperature ( T x ), showing normal thermal expansion behaviour [31] , [32] , [33] . We used the 1/3 power law function between the volume and Q 1 , ( V ) 1/3 ~( d )~1/ Q , to estimate the volume contraction roughly, and found it was around 1.3% (the fractal law yielded a volume contraction of 1%). Note that changing the temperature from 293 to 390 K, the power exponent could alter a bit (while the trend of ‘larger Q 1 , smaller volume’ works at both temperatures), and the precise relationship between the local volume change (determined from Q 1 ) on medium-range length scale and the microscopic volume change near T g remains to be settled in the future. Accompanying the NTE, local ordering and rearrangement of the MRO and SRO occur obviously as seen from the temperature dependence of Q 2 /Q 1 and the full width at half maximum of Q 1 ( Fig. 1d ). The abnormal NTE observed here implies unique SRO and MRO structures of Ce-MG, which supports the highly unusual anharmonic vibrational modes. Furthermore, from the in situ synchrotron XRD measurements under high pressures at 390 K, we find that the NTE occurs over a wide pressure range, while under higher pressures (above 20 GPa) normal thermal expansion restores. We will discuss the near- T g behaviours and the possible structural origins of NTE below. 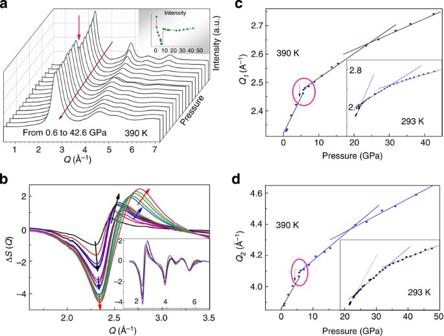Figure 2: Structure change with pressure measured at 390 K. (a)In situXRD patterns of the Ce65Al10Co25MG under high pressure from 0.6 to 42.6 GPa at 390 K. The inset shows the pressure dependence of the diffraction intensity. (b) The difference plot ofΔS(Q)−QaroundQ1and for the wholeQrange measured (the inset) for Ce65Al10Co25MG at 390 K. (c) Pressure dependence ofQ1at 390 and 293 K (the inset). (d) Pressure dependence ofQ2at 390 and 293 K (the inset). The straight lines are used as a guide to distinguish the different amorphous states. Error bars incandd, which are smaller than the symbol size represent the accuracy ofQ1andQ2detemined from the fitting. Structure evolution at 390 K Figure 2a shows the XRD patterns recorded at 390 K under different pressures. No sharp Bragg peaks are observed and only the amorphous diffraction maxima change their intensity in the entire pressure range, which implies that the glassy structure is rather stable upon compression even near T g . Same with the behaviour at 293 K, the diffraction intensity maxima in the regions of 3.0–4.5 Å −1 and 5.0–6.5 Å −1 diminished gradually with increasing pressure (the 5.0–6.5 Å −1 feature almost disappear finally). However, the intensity of the maximum between 4.0 and 5.5 Å −1 diminished gradually with increasing pressure, which is different from the intensified behaviour between 4.0 and 5.5 Å −1 at 293 K. A quantitative analysis of the pressure dependence of Q 1 and Q 2 ( Fig. 2 ) indicates a multi-densification process at both 293 and 390 K. Accordingly, the amorphous phase can be divided into low-, medium- and high-density amorphous states (referred as LDAS, MDAS and HDAS, respectively) with distinct compressibilities. As seen from Fig. 2b , the multiple transformations can be further indicated by the change of the total structure factors with the applied pressures: ΔS p ( Q )= S p ( Q )− S 0.6 GPa ( Q ). Changing the temperature from 293 to 390 K increases the transformation pressures from ~4.4 to ~5.5 GPa for the LDAS–MDAS transformation, and from ~23.3 to ~25.3 GPa for the MDAS–HDAS transformation. Another significant observation here is that, in contrast with the smooth change from LDAS to MDAS at 293 K (the inset of Fig. 2c ), a relatively sharp and discontinuous change of Q 1 is observed around 5.5 GPa for the sample measured at 390 K as seen in Fig. 2c . The continuous and discontinuous transformation at 293 and 390 K can be seen more clearly in Fig. 3a . At 390 K, the volume change (according to the 1/3 power law) around the LDAS–MDAS transformation is around 1.8% between 5.5 and 5.7 GPa (the volume collapse is ~1.2% around 5.5 GPa after extrapolation). We should stress that the volume collapse of ~1.2% is large enough to render a structure transformation, since the volume difference between a bulk MG and its fully crystallized counterpart is usually ~0.3–1.0%. Similar discontinuous change can also be observed from the pressure dependence of Q 2 ( Fig. 2d ), and the diffraction intensity shows an abrupt change as well around 5.7 GPa (the inset of Fig. 2a ). As seen from the inset of Fig. 2a , the diffraction intensity decreases with increasing pressure rapidly in the LDAS, after obtaining an abrupt increase, decreases slightly in the MDAS (5.7–25 GPa) and increases slightly in the HDAS. Note that at RT (near T g ) the continuous (discontinuous) transformation occurs around 4.4 Gpa (5.5 GPa), which is similar to the upper end of the polyamorphic transformation range of 1.5–5.0 GPa for Ce 75 Al 25 MG [29] . Figure 2: Structure change with pressure measured at 390 K. ( a ) In situ XRD patterns of the Ce 65 Al 10 Co 25 MG under high pressure from 0.6 to 42.6 GPa at 390 K. The inset shows the pressure dependence of the diffraction intensity. ( b ) The difference plot of ΔS ( Q )− Q around Q 1 and for the whole Q range measured (the inset) for Ce 65 Al 10 Co 25 MG at 390 K. ( c ) Pressure dependence of Q 1 at 390 and 293 K (the inset). ( d ) Pressure dependence of Q 2 at 390 and 293 K (the inset). The straight lines are used as a guide to distinguish the different amorphous states. Error bars in c and d , which are smaller than the symbol size represent the accuracy of Q 1 and Q 2 detemined from the fitting. 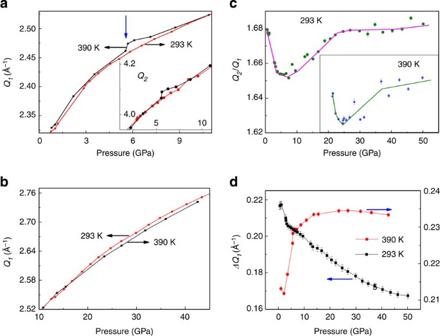Figure 3: Pressure-induced structure changes measured at 293 and 390 K. (a) Pressure dependence ofQ1andQ2(the inset) below 10 GPa measured at 293 and 390 K. (b) Pressure dependence ofQ1above 10 GPa measured at 293 and 390 K. (c) Pressure dependence ofQ2/Q1at 293 and 390 K (the inset). (d) Pressure dependence of the full width at half maximum ofQ1at 293 and 390 K. Error bars, representing the accuracy ofQ1andQ2detemined from the fitting, are given ina-d. Full size image Figure 3: Pressure-induced structure changes measured at 293 and 390 K. ( a ) Pressure dependence of Q 1 and Q 2 (the inset) below 10 GPa measured at 293 and 390 K. ( b ) Pressure dependence of Q 1 above 10 GPa measured at 293 and 390 K. ( c ) Pressure dependence of Q 2 / Q 1 at 293 and 390 K (the inset). ( d ) Pressure dependence of the full width at half maximum of Q 1 at 293 and 390 K. Error bars, representing the accuracy of Q 1 and Q 2 detemined from the fitting, are given in a - d . Full size image Furthermore, it is clearl from the figure that below 9.0 GPa, the Q 1 obtained at 390 K locates above that obtained at 293 K under a given pressure, indicating the occurrence of NTE in the range of 0.6–9 GPa. The largest NTE after heating from RT to 390 K occurs around 5.7–5.5 GPa, where the relative volume contraction is around 2%. Between around 9.0 and 20 GPa, the two curves nearly overlap together, suggesting roughly zero (or very small) thermal expansion. However, above 20 GPa, the Q 1 obtained at 390 K locates below that obtained at 293 K under a given pressure, indicating a normal thermal expansion behaviour. Usually the vibrations of atoms increase with increasing temperature, which leads to an increase of the average bond distance due to the asymmetry of the potential well. However, NTE can be observed in some classes of materials with open/flexible structures and/or ferromagnetic or ferroelectric microdomains. For a large number of NTE materials, such as the zirconium tungstate family, scandium tungstate family, zeolites and aluminium phosphates [34] , [35] , [36] , the NTE can be described in the framework of ‘rigid unit modes’ associated with concerted tilting or rocking motions of rigid polyhedra (MO 4 tetrahedra or MO 6 octahedra) when transverse vibrations of the corner-sharing oxygen atoms are excited [34] , [35] , [36] , [37] . Since there are no open structures or magnetic domains present in an MG with a densely packed structure, the NTE observed here is unusual, which could be related to the weakly bonded linkage-atom zones, providing space and flexibility for the relaxation/rearrangement of the tightly bonded SSCs. Here, we argue that the multiple-densification processes with/without a discontinuous volume change, along with the NTE behaviour, can be understood from the transformations and relaxations of the hierarchical configurations including weakly bonded zones and tightly bonded SSCs. Despite the still elusive disordered structure, MGs are well known to have some degree of SRO, characterized by SCCs, and MRO constructed by geometric/topological packing of the SRO clusters [38] , [39] . Several building schemes, such as face-centred cubic packing, hexagonal close-packed packing, icosahedral(-like) ordering and so on were proposed, and the fractal characteristic of MRO was revealed [30] , [38] , [39] , [40] . For Ce 65 Co 25 Al 10 MG, there are Co-centred clusters and Al-centred clusters (marked as S in the inset of Fig. 1c ), each of which is made up of a solute atom surrounded by a majority of solvent Ce atoms. Considering a large concentration of Co, two Co atoms can form an isolated pair surrounded by Ce atoms, causing the formation of extended clusters (marked as E in the inset of Fig. 1c ). Al–Co pair-centred extended cluster is also possible due to their strong interaction with covalent bonding-like characteristics [41] . Even the solute–solute connection (Al–Al or Co–Co or Al–Co) could become network-like due to a high concentration (35%) of Al and Co. The icosohedral-like and/or crystal-like ordering of the nearest-neighbour SCCs (type S) constitute the main MRO through inter-cluster Ce–Ce bonding [38] , [39] . Other types of MRO include network-like superclusters and the dense packing of the extended clusters via edge-, vertex- or face-sharing [38] , [39] . Besides, there are loosely packed solvent Ce atoms among the tightly bonded SSCs, and these linkage atoms are characterized mainly by weak Ce–Ce bonding. The hierarchical bonding nature thus can be illustrated from the above model. The SCCs can be considered a rigid unit (or molecule) at certain temperature and pressure ranges due to the strong solute–solvent bonds (Ce–Al and Ce–Co) within the clusters, while the Ce-rich linkage atoms constitute the weakest bonding zones. And the inter-cluster Ce–Ce bonds, which connect nearest-neighbour SCCs to form icosohedral-like and/or crystal-like order, possess the medium strength of interaction. Under pressure, it is reasonable to speculate that the Ce atoms associated with these Ce-rich linkage atoms are preferentially strained to accommodate the applied pressure, and the inter-cluster Ce–Ce bonds begin to shorten and tilt gradually without significant change of the SCCs themselves (as seen from the sketch map in Fig. 4a ). The LDAS to MDAS transformation is thus mainly due to the shortening of the weak Ce–Ce bonds among SCCs (including the the weak Ce–Ce bonds among the linkage atoms and inter-cluster Ce–Ce bonds), which can be promoted by the delocalization of 4 f electrons. It should be stressed that during this stage when the pressure is not large enough, slight rotation/distortion is possible, but its contribution to the volume reduction can be neglected. These relatively weak bonds among the tightly bonded SSCs become rigid gradually with increasing pressure. When the strength of these initially weak bonds among the SCCs approaches those of the Ce–Ce/Ce–Al(Co) bonds within SCCs, further increasing the pressure will make the SCC shrink and the polyhedral cluster distort ( Fig. 4a ). The gradual MDAS to HDAS transformation thus indicates substantial shrinkage and distortion of the SCCs (related to all Ce–Al, Ce–Co and Ce–Ce bonds of SCCs). The hierarchical densification nature can be further revealed from the pressure dependence of Q 2 /Q 1 ( Fig. 3c ), which shows different changes in the LDAS, MDAS and HDAS, implying distinct densification mechanisms associated with different degrees of change of the linkage-atom zones, SRO and MRO. The scattered intensity of a glass, I ( q ), can be calculated by the Debye formula, I ( q )=∑ f i f j sin ( qr ij )/ qr ij , where r ij is the interatomic distance between atoms j and i, and f i is the atom form factor. If all interatomic distances r ij decreases with pressure by the same factor r ij ( P )= r ij (1+ a*P )= r ij * k , the scattered intensity I ′( q / k ) is equal to I ( q ). This means that the ratio of any diffraction maxima positions is constant for different pressures. As seen from Fig. 3c , the deviation of Q 2 /Q 1 from a constant value clearly indicates the ongoing hierarchical change of the MRO and SRO with pressure. It is generally accept that the Q 1 reflects the MRO correlation in real space, while the high- Q peaks reflect the SRO features. Following this tendency, the Q 1 and Q 2 can be considered to reflect roughly the change of the local structure on larger- and shorter-length scales, respectively. From the figure, the decrease of Q 2 /Q 1 with increasing pressure in LDAS indicates that a larger structure change occurs on a larger-length scale, and the opposite behaviour is observed in the MDAS. In contrast, approaching a constant value of Q 2 /Q 1 in the HDAS suggests that pressure degrades the hierarchical bonds nature significantly in this high pressure range, where the amorphous structure is pressurized in a more homogeneous way (all interatomic distances tend to decrease with pressure by a similar factor) like an isotropic crystalline solid. In addition, the above multiple-densification process implies that a totally new amorphous phase and even devitrification may emerge above the second-stage transformation pressure in REMGs, where significant change of SCCs occurs. Recently, the pressure-induced devitrification in Ce 75 Al 25 MG was reported [29] , where the transformation pressure of around 25.3 GPa is remarkably similar to the intersection point of the MDAS and HDAS (23 GPa) in our alloy. In the present alloy, the shrinkage and distortion of the SCCs result in MDAS–HDAS transformation instead of devitrification because of the composition effect [13] and especially the Co addition (which enhances the frustration to impede devitrification and render partial delocalization of 4 f electrons). 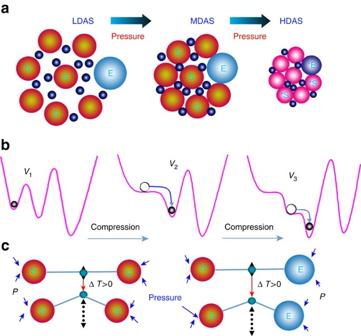Figure 4: Schematic maps showing the structural and dynamical changes. (a) Illustration of hierarchical densification of Ce65Al10Co25metallic glass. The smallest cyan ball represents the Ce atom, the medium-sized colour (orange and blue) ball represents the solute-centred cluster (S) and the largest colour (orange and blue) ball represents the supercluster (E). During the LDAS–MDAS transformation, the SCCs remain largely unchanged and primarily the weak Ce–Ce bonds among the tightly SCCs shorten significantly. During the MDAS–HDAS transformation, not only the initially weak bonds among SCCs stiffen, but also the SCCs shrink and/or distort significantly (as illustrated from the smaller size and different colours of the SCCs: from E to *E, and S to *S). (b) Schematic representation of the pressure-induced mechanical instabilities in metallic glasses. The curves represent the potential energy along the relevant coordinate, at a given volume ofV1,V2orV3(V1>V2>V3); the circles represent the position of the system. (c) Schematics of relaxation and vibrational modes leading to NTE: relaxation with the aid of transverse vibrational motion of sharing the Ce atom in a SCC–Ce–SCC linkage causing a decrease of the SCC–SCC distance (other contribution may come from the cooperative rocking and/or tilting motions of the neighbouring SSCs). The arrows indicate the influence of external pressure on the relaxation and vibrational motions. Figure 4: Schematic maps showing the structural and dynamical changes. ( a ) Illustration of hierarchical densification of Ce 65 Al 10 Co 25 metallic glass. The smallest cyan ball represents the Ce atom, the medium-sized colour (orange and blue) ball represents the solute-centred cluster (S) and the largest colour (orange and blue) ball represents the supercluster (E). During the LDAS–MDAS transformation, the SCCs remain largely unchanged and primarily the weak Ce–Ce bonds among the tightly SCCs shorten significantly. During the MDAS–HDAS transformation, not only the initially weak bonds among SCCs stiffen, but also the SCCs shrink and/or distort significantly (as illustrated from the smaller size and different colours of the SCCs: from E to *E, and S to *S). ( b ) Schematic representation of the pressure-induced mechanical instabilities in metallic glasses. The curves represent the potential energy along the relevant coordinate, at a given volume of V 1 , V 2 or V 3 ( V 1 > V 2 > V 3 ); the circles represent the position of the system. ( c ) Schematics of relaxation and vibrational modes leading to NTE: relaxation with the aid of transverse vibrational motion of sharing the Ce atom in a SCC–Ce–SCC linkage causing a decrease of the SCC–SCC distance (other contribution may come from the cooperative rocking and/or tilting motions of the neighbouring SSCs). The arrows indicate the influence of external pressure on the relaxation and vibrational motions. Full size image From the point of view of energy landscape, the LDAS, MDAS and HDAS correspond to the distinct megabasins on the potential energy surface. Since there are energy barriers among the megabasins, thermal activation is needed to cause a structural transformation. Therefore, the polyamorphic transformation could be kinetically hindered at low temperatures. And the LDAS can persist until an external pressure-induced local mechanical instability occurs. Therefore, the LDAS–MDAS and MDAS–HDAS transformations in present alloy occur by gradual spinodal decomposition at different pressures as illustrated in Fig. 4b . Well below T g , such local mechanical instability occurs over a broad pressure range due to the variety of local structures in the glass, resulting in a continuous transformation from LDAS to MDAS (as observed by other authors). Around T g , the accelerated kinetics and the narrowed distribution of local environments manifest the hidden first-order-like transformation, as implied from the relatively discontinuous volume change in the present alloy. Such a discontinuous change is not expected to occur for a second-order transformation. However, the MDAS–HDAS transformation is always smooth and continuous at both RT and 390 K ( Fig. 2c,d ), different from the LDAS–MDAS transformation, which implies their different transformation types in nature (first-order LDAS–MDAS and second-order MDAS–HDAS transformations). In addition to the difference of continuous vs discontinuous change around the LDAS–MDAS transformation, the peak-shape change of the diffraction patterns under high pressure further reveals the different local structure arrangements at RT and 390 K. Figure 3d compares pressure dependence of the full width at half maximum of FSDP of the XRD patterns recorded at 293 and 390 K. The FSDP of the RT patterns sharpens rapidly during the initial pressure range below 4.0 GPa, then slows down its pace gradually and approaches to a constant value above 45.0 GPa. In contrast, the FSDP of the near- T g patterns broaden rapidly below 6.0 GPa after an initial rapid sharpening, then slows down its pace gradually between 6.0–14.0 GPa, and retains nearly a constant value above 14 GPa. Since the FSDP correlates with the MRO, the sharpening of the FSDP implies that the correlation length becomes longer and the structure becomes more ordered on the medium-range scale with increasing pressure at RT. Near T g , the structure has already become more ordered and the density of the liquid-like atomic sites increases significantly as a precursor for glass transition. The broadening of the FSDP with increasing pressure suggests the stiffening of these liquid-like bonds and disordering of the locally ordered structures. The NTE of the Ce-based MG can be illustrated based on the above weakly bonded linkage atoms plus SSCs’ configuration. One probable contribution to the NTE may come from the relaxation of the intermediate-range structure under pressure. To further check the structure relaxation effect on the NTE behaviour and the first-order-like LDAS–MDAS transformation, we carried out time-dependent experiments at 390 K under fixed pressure ( Fig. 5a ). First we set the pressure at 6.21 GPa at RT, and then we increased the temperature gradually to 390 K (see the Methods and also ref. 42 ). When approaching and stabilizing the temperature at 390 K, the pressure first increased a little to 6.27 GPa and decreased gradually and finally stabilized around 6.05–6.01 GPa. The first pressure point locating within 6.05–6.01 GPa was chosen as the base point, and the evolution of diffraction patterns with time was recorded. Under a pressure of ~6 GPa, the glass is finishing the LDAS–MDAS transformation, therefore, the initial glass for relaxation experiments is nearly in the unrelaxed MDMS form. As seen in Fig. 5a , the XRD patterns show almost the same features with a broad hump around 2.5 Å −1 and two diffraction Au peaks (as a pressure calibrant), and Q 1 increases slightly with increasing time. Within 120 min, the relaxation results in a volume reduction of ~0.2%, which is much smaller than the volume collapse of 1.2% around 5.5 GPa and the volume change of ~1.8% between 5.5 and 5.7 GPa at 390 K ( Fig. 3a ). This large difference further indicates that the pressure-induced first-order-like LDAS–MDAS transformation near T g does not arise from the relaxation effect. The volume contraction of 2% (around 5.5–5.7 GPa) after heating the sample from RT to 390 K is also much larger than the relaxation effect of 0.1–0.3%. This indicates that in addition to the less-important relaxation effect, other local atomic arrangement mechanisms are involved for the NTE behaviour. Note that the timescale of our relaxation experiments is much longer (120 min) than the X-ray exposure time (1–3 min) and the time interval (around 12 min) between two neighbouring collections. Therefore, the practical relaxation effect during our high-pressure experiments is even much smaller than the relaxation experiments. 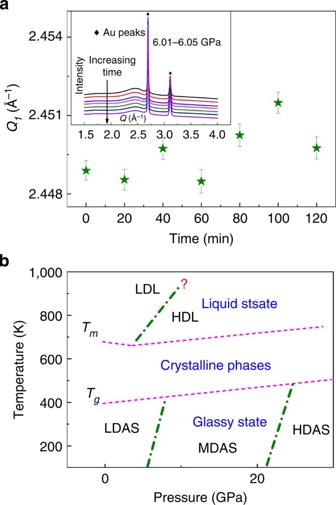Figure 5: Relaxation behaviour and the schematic phase diagram. (a) Time dependence ofQ1measured under fixed pressure (around 6.03 GPa) and temperature (390 K). Error bars, representing the accuracy ofQ1detemined from the fitting, are shown. The inset shows theIn situXRD patterns of the Ce65Al10Co25MG recorded at different time under ~6.03 GPa. (b) Schematic pressure–temperature phase diagram of Ce65Al10Co25metallic glass.Tmis the melting temperature,Tgis the glass transition temperature. LDL and HDL stand for the possible low-density and high-density liquid states, respectively. The question mark indicates that the existence of LDL–HDL transition is speculative. Figure 5: Relaxation behaviour and the schematic phase diagram. ( a ) Time dependence of Q 1 measured under fixed pressure (around 6.03 GPa) and temperature (390 K). Error bars, representing the accuracy of Q 1 detemined from the fitting, are shown. The inset shows the In situ XRD patterns of the Ce 65 Al 10 Co 25 MG recorded at different time under ~6.03 GPa. ( b ) Schematic pressure–temperature phase diagram of Ce 65 Al 10 Co 25 metallic glass. T m is the melting temperature, T g is the glass transition temperature. LDL and HDL stand for the possible low-density and high-density liquid states, respectively. The question mark indicates that the existence of LDL–HDL transition is speculative. Full size image From the hierarchical configuration of MG, we argue that the NTE could be related to the tilting or rocking motions of the neighbouring SCCs (besides the relaxation effect), which tend to pull the neighbouring SCCs towards each other. This kind of motion could be seen more locally as the flexing of the SSC–junction (atom)–SCC chains through transverse motions of the sharing vertex-Ce atom or other junction atom (see Fig. 4c ). These low-energy vibrations are similar to the rigid unit modes of ZrW 2 O 8 showing NTE behaviour, which involve the transverse vibrational motion of an oxygen atom in a M–O–M linkage and the collective rocking of the rigid ZrO 6 octahedra [35] . Increasing the temperature will accelerate the vibration of the linkage atoms, and thus promote the collective tilting or rocking of the polyhedra, resulting in an increasing densification pace with increasing temperature ( Fig. 1c ). The change of the local structures induced by relaxation and the above motions can be further revealed from the temperature dependence of Q 2 /Q 1 under 0.6 GPa ( Fig. 1d ). Above 370 K, the Q 2 /Q 1 decreases with increasing temperature rapidly, which is contrary to the gradual increase of Q 2 /Q 1 upon increasing temperature in a Pd-based bulk metallic glass (BMG) showing normal thermal expansion [31] , [33] . The decrease of Q 2 /Q 1 with increasing temperature is similar to the pressure effect in the low-pressure range, indicating that the temperature-induced structure change under 0.6 GPa mainly occurs on the MRO scale. The above-mentioned low-energy vibrational motions is supported by the unique anharmonic potential well of Ce-based MGs. From an acoustic investigation under a pressure range of 0–0.5 GPa, it was found out that γ l (longitudinal Gruneisen parameter) of a Ce-based MG was negative, different from the positive γ l in other MGs, but similar to SiO 2 glass [43] , [44] . Since normally a necessary condition for the occurrence of NTE is the presence of low-energy phonons with negative γ i values, the existence of highly anharmonic long-wavelength vibrational modes with negative γ l and γ a indicates the possibility of NTE in a certain temperature–pressure window. Under higher pressure (above 20 GPa), the rigid unit modes associated with polyhedral clusters tend to vanish, since the weak bonds linking the clusters have already become stiff and because of much less free volume left, making relaxation and tilting/rocking motions of the SCCs and transverse motions of the junction atoms more difficult. Note that a similar densification effect with increasing temperature under a certain pressure range was also observed experimentally in silica glass, which was related to a redistribution of the ring size and a collapse of void space [25] . The above investigations indicate that the structural polyamorphousim and dynamics under high pressure and/or high temperature are remarkably plentiful in MG systems. Due to the inherent structural inhomogeneity and the dispersion of the bonding features on the scales smaller than the correlation length of MRO, which are general features of MGs [30] , [38] , [39] , [40] , [45] , [46] , pressure essentially modifies the medium-to-short-range order and densifies the amorphous structure hierarchically in all MG systems. Owing to the special 4 f electron delocalization, which assists largely in the bond shortening, the multiple densifications are easy to recognize in Ce-based MGs. The LDAS–MDAS transformation, observed here, which primarily is related to the shortening of the weak Ce–Ce bonds among the SSCs and does not undergo significant change in SRO, is similar to the first-order isostructural γ–α transition of pure Ce (where the SRO of unit cell remains face-centred cubic). In contrast, the MDAS–HDAS transformation, associated with the change of SRO, is somehow similar to the normal polymorphic transition in crystals involving a distinct change of SRO in the unit cell. The change of the SCCs also implies that the hierarchical interactions can be significantly degraded under high pressure, since all the bonds within and among the SCCs tend to approach the same level of strength above a certain threshold pressure. The pressure-induced change of the hierarchical bonding, as revealed in this study, will exert significant impacts on the mechanical, dynamics and glass transition of various MG systems, due to their strong dependence on both the SRO, MRO and linkage-atom (free volume) zones [15] , [16] , [17] , [45] , [46] , [47] , [48] . These issues are remaining to be settled. In addition, it is well known that the polyamorphsim of glassy or amorphous solids mimics (usually is not mapped onto) the density-driven liquid–liquid phase transition in the corresponding liquids (if there exists). However, at present the knowledge about the structure evolution of MG-forming liquids under high pressure is little explored and rather poorly understood. Recently, the existence of a first-order liquid–liquid phase transition in the monatomic liquid Ce metal has been experimentally testified, which primarily arises from the f electron delocalization [49] . Glass is usually considered as a frozen liquid, thus near T g a glass inherits and manifests mostly the corresponding liquid features. Thus, the first-order-like LDAS–MDAS transformation near T g in Ce-based MG may be mapped onto an underlying first-order liquid–liquid phase transition of its corresponding liquids driven by entropy contrasts. Figure 5b presents a schematic phase diagram of the Ce-based MG. The existences of a low-density liquid–high-density liquid transition line with a positive Clapeyron slope (see Fig. 5b ) and a minimum of the melting temperature are speculative based on a combination of the present observations and the high-pressure behaviours of liquid Ce metal. Experimentally, it is to be clarified in the future whether the critical point (if there is) locates above the melting point, or the low-density liquid–high-density liquid transition occurs in the supercooled liquid state such as H 2 O. Our findings may shed light on the nature of the near- T g polyamorphic transformations of the MG system, and bear important implications on the hierarchical structural process under extreme conditions (high pressure and/or high temperature) in glassy metals and the corresponding liquids. Sample preparation First a master alloy ingot was prepared by arc melting pure Ce, Al and Co in a Ti-gettered argon atmosphere. The ingot was remelted several times for homogeneity. Then the Ce-based MG ribbon was prepared by single-roller melt-spinning technique using the ingot. High-pressure synchrotron X-ray measurements The in situ high-pressure synchrotron X-ray measurements with a focused X-ray beam of 15 × 15 μm 2 at a wavelength of 0.3738 Å were performed at Beamline ID27 of the European Synchrotron Radiation Facilities in Grenoble, France. The pressure was generated using a DAC with the culet of 400 μm in diameter. The sample was cut and ground into small chips, and then was loaded into the DAC along with the pressure-calibrator ruby. Helium was used as the pressure-transmitting media, which could provide the best hydrostatic condition to pressures above 100 GPa. MAR 345 image plate detector was used to collect the diffraction signal, and the XRD patterns were integrated from the images using the FIT2D software. The structure factors of the sample were obtained using the PDFgetX2 software. High-temperature relaxation experiments The relaxation experiments under fixed pressure and temperature were carried out at Beamline 4W2 of the Beijing Synchrotron Radiation Facilities in Beijing, China. The incident X-ray beam was monochromatized to a wavelength of 0.6199 Å. The doubly focused X-ray beam size was 35 × 12 mm 2 . A 4:1 mixture of ethanol–methanol was used as pressure-transmitting medium, and for pressure calibration Au powders were dispersed inside. The pressure applied to the sample was calculated from the lattice constant of Au using the equation of state of Au. A resistance-heating system (ref. 42 ) was used to heat the sample in DAC, and temperature was measured by the NiCr–NiSi thermocouple with its precision <±1 °C. How to cite this article: Luo, Q. et al. Hierarchical densification and negative thermal expansion under high pressure in Ce-based metallic glass. Nat. Commun. 6:5703 doi: 10.1038/ncomms6703 (2015).